RHOA inactivation enhances Wnt signalling and promotes colorectal cancer Activation of the small GTPase RHOA has strong oncogenic effects in many tumour types, although its role in colorectal cancer remains unclear. Here we show that RHOA inactivation contributes to colorectal cancer progression/metastasis, largely through the activation of Wnt/β-catenin signalling. RhoA inactivation in the murine intestine accelerates the tumorigenic process and in human colon cancer cells leads to the redistribution of β-catenin from the membrane to the nucleus and enhanced Wnt/β-catenin signalling, resulting in increased proliferation, invasion and de-differentiation. In mice, RHOA inactivation contributes to colon cancer metastasis and reduced RHOA levels were observed at metastatic sites compared with primary human colon tumours. Therefore, we have identified a new mechanism of activation of Wnt/β-catenin signalling and characterized the role of RHOA as a novel tumour suppressor in colorectal cancer. These results constitute a shift from the current paradigm and demonstrate that RHO GTPases can suppress tumour progression and metastasis. The strong oncogenic role of small GTPases was first realized over three decades ago, when activation of the rat sarcoma oncogene homolog (RAS) was shown to be an important event in the tumorigenic process [1] , [2] . GTPases function as molecular switches cycling between a GTP-bound active form and an inactive GDP-bound form. In the GTP-bound state they are able to interact with effector or target molecules to initiate a downstream response, while their intrinsic GTPase activity returns the proteins to the GDP-bound state, to complete the cycle and terminate signal transduction [3] , [4] . The activation state of GTPase proteins is regulated by three kinds of regulators: guanine nucleotide exchange factors, which promote the exchange of GDP for GTP; GTPase activating proteins, which enhance the intrinsic GTPase activities of Rho GTPases; and Rho GDP dissociation inhibitors, which interact with GDP-bound Rho GTPases and sequester them from the membrane to the cytoplasm. The RHO (Ras homology) subfamily of GTPases includes more than 20 members, represented by the canonical proteins RHOA, RAC1 and CDC42, which have long been known to regulate the structure of the actin cytoskeleton as well as proliferation, differentiation, migration and polarity of epithelial cells [5] , [6] , [7] . Therefore, it is not surprising that RHO GTPase signalling cascades are commonly deregulated during tumorigenesis. The vast majority of the data currently available regarding the role of RHO GTPases in cancer indicate that these proteins are frequently overexpressed and/or activated, significantly contributing to tumour progression in multiple tissues [8] , [9] . Although RHOA activation does not transform fibroblasts, it strongly cooperates with RAS to induce transformation [10] , and participates in the key aspects of the oncogenic process such as proliferation, polarization, apoptosis, adhesion, migration, invasion and metastasis [5] , [11] , [12] , [13] , [14] , [15] . Colorectal cancer is one of the leading causes of cancer-related death in the Western World [16] . In normal intestinal epithelial cells, canonical Wnt signalling is important to maintain a proliferative compartment and is initiated by the interaction of Wnt ligands and Frizzled receptors. This results in the stabilization of β-catenin, which then accumulates in the cytoplasm and translocates to the nucleus, where it binds to T-cell factor/lymphoid enhancer factor (TCF/LEF) transcription factors and regulates the expression of the key cell cycle regulators such as c-MYC or Cyclin D1 (refs 17 , 18 ). Constitutive hyperactivation of canonical Wnt signalling is a major hallmark of colorectal cancer and is associated with APC mutations in >70% of the sporadic cases [19] . RHOA has been shown to be an important mediator of the noncanonical Wnt/planar cell polarity (PCP) pathway, a signalling cascade initiated also by Wnt ligands binding to Frizzled/LRP receptors, but that does not signal through TCF4/β-catenin [20] . Although earlier studies have shown that the noncanonical Wnt5a ligand can regulate the motility of colon cancer cells, the role of RHOA in this process has not been investigated and Wnt5a overexpression had no effects in a mouse model of intestinal tumorigenesis ( Apc 1638N mice) [21] . On the other hand, the role of RHOA in the canonical Wnt signalling pathway and in the progression of colorectal tumours is poorly characterized and comprehensive studies using animal models are currently lacking. The RHO activator lysophosphatidic acid (LPA) has been reported to activate TCF4/β-catenin activity, increase proliferation [22] and prevent apoptosis [23] in colon cancer cell lines. Moreover, in a rat model of colorectal cancer, LPA resulted in the activation of RHOA and significantly increased metastasis [24] . However, LPA has multiple effects mediated by different receptors and it is not clear to what extent the observed responses to LPA are mediated by RHO proteins [25] . It has been shown that RHOA is overexpressed in colorectal tumours [26] and RHOA silencing was reported to suppress the growth of colon cancer xenografts in immunodeficient mice [27] . However, we have shown that reduced RHOA levels in colorectal tumours are associated with poor patient prognosis [28] and transforming growth factor-β-induced epithelial-to-mesenchymal transition has been shown to be associated with reduced RHOA activity [29] , [30] . Here we used mouse models of genetic and carcinogen-induced intestinal carcinogenesis to demonstrate that reduced RhoA activity in the intestine significantly accelerates the tumorigenic process, resulting in shorter animal survival and increased tumour size and multiplicity. We then used in vitro models to demonstrate that in colon cancer cells, the loss of RHOA is associated with increased proliferation, tumour growth and motility/invasion as well as reduced differentiation. Moreover, reduced RHOA levels were observed in metastatic sites compared with paired primary human tumours, and targeted inactivation of RHOA resulted in increased lung metastasis in a mouse model. Importantly, we found that RHOA inactivation results in the accumulation of nuclear β-catenin and increased TCF4/β-catenin activity. Collectively, our results demonstrate that the loss of RHOA significantly contributes to the progression of colorectal tumours through the activation of canonical Wnt signalling. RHOA inactivation accelerates intestinal tumorigenesis We have previously reported that reduced RHOA tumour levels are associated with poor prognosis of colorectal cancer patients [28] . However, it is currently not known whether RHOA directly modulates the progression of colorectal tumours. Here we generated mice with targeted inactivation of RhoA in the intestinal epithelium by crossing mice with Cre-dependent expression of a thoroughly characterized dominant negative form of RhoA (N19; RhoA DN ) [10] , [31] , [32] with mice expressing Cre recombinase under the control of the intestine-specific Villin 1 promoter ( Vil-Cre TG ; Supplementary Fig. 1a ). Dominant negative RhoA expression and reduced RhoA activity were confirmed in intestinal epithelial cells of the compound transgenic mice ( Vil-Cre TG/− ;RhoA DN/− ) compared with control mice ( Cre −/− ;RhoA DN/− ; Supplementary Fig. 1b–d ). The Apc min/+ mouse model carrying heterozygous mutations of the tumour-suppressor gene Apc was used to initiate intestinal tumorigenesis as previously described [33] , [34] . Inactivation of RhoA in the intestine of Apc min mice ( Apc min/+ ;Vil-Cre TG/− ;RhoA DN/− ) resulted in a significant reduction of their survival compared with control animals ( Apc min/+ ;Vil-Cre −/− ;RhoA DN/− ; Fig. 1a ). Consistently, 13-week-old animals with intestinal inactivation of RhoA had significantly more tumours in their small intestine ( Fig. 1b,c and Supplementary Fig. 2a,b ), which were significantly larger than in the control mice ( Fig. 1d ). Moreover, a significant increase in the number of proliferating cells (bromodeoxyuridine (BrdU)-positive) was observed in the intestinal tumours derived from RhoA-dominant negative mice compared with control mice ( Fig. 1g–i ), likely explaining the larger tumour size observed in the RhoA DN mice. As an alternative mechanism of tumour initiation, we used azoxymethane (AOM), an intestinal-specific chemical carcinogen. Consistent with the findings obtained using the Apc min model, reduced RhoA activity in the Vil-Cre TG/− ;RhoA DN/− mice resulted in a significant increase in the number of small intestinal tumours after AOM treatment compared with control Vil-Cre −/− ;RhoA DN/− animals ( Fig. 1e ), although there was no difference in the size of these tumours ( Fig. 1f ). No differences were observed in the number and size of tumours in the large intestine initiated genetically or pharmacologically ( Supplementary Fig. 2c–f ). Collectively, these results demonstrate that the downregulation of RhoA activity is an important event contributing to intestinal tumour progression. 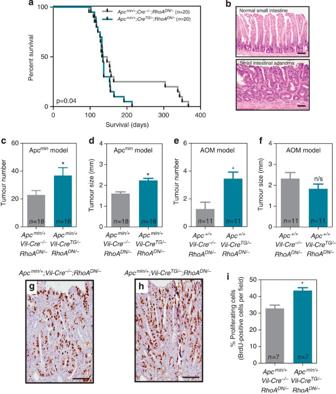Figure 1: Effects of RhoA inactivation on intestinal tumorigenesisin vivo. (a) Lifespan of mice with heterozygous mutations of the tumour suppressor geneApc(Apcmin/+) with normal intestinal levels of RhoA (Apcmin/−;Vil-Cre−/−;RhoADN/−) or RhoA inhibition due to forced expression of DN-RhoA (Apcmin/−;Vil-CreTG/−;RhoADN/−). (b) Representative histology of the normal small intestine and intestinal adenomas. The average number (c) and size (d) of macroscopic tumours observed in the small intestine of 13-week-oldApcmin/−;Vil-CreTG/−;RhoADN/−animals and controlApcmin/−;Vil-Cre−/−;RhoADN/−mice are shown (n=18). The average number (e) and size (f) of small intestinal tumours induced by AOM treatment inVil-Cre−/−;RhoADN/−animals andVil-CreTG/−;RhoADN/−mice are shown. (g,h) Mice were i.p. injected with 100 mg kg−1BrdU 2 h before being killed. The number of cells in the S-phase of the cycle during this time was assessed with anti-BrdU immunohistochemistry. (i) Pictures were taken under a bright-field microscope at × 20 and the number of proliferative cells in the small intestinal tumours of DN-RhoA (Apcmin/+;Vil-CreTG/−;RhoADN/−) and control (Apcmin/+;Vil-Cre−/−;RhoADN/−) mice was quantified blinded from the animal identity. At least 1,000 total tumour cells were scored per mouse and there were seven mice per group.N: number of animals per group. The mean (±s.e.m.) is shown. *Student’st-testP<0.05; n/s: not significant. Scale bars, 100 μm. Figure 1: Effects of RhoA inactivation on intestinal tumorigenesis in vivo. ( a ) Lifespan of mice with heterozygous mutations of the tumour suppressor gene Apc ( Apc min/+ ) with normal intestinal levels of RhoA ( Apc min/− ; Vil-Cre −/− ; RhoA DN/− ) or RhoA inhibition due to forced expression of DN-RhoA ( Apc min/− ; Vil-Cre TG/− ; RhoA DN/− ). ( b ) Representative histology of the normal small intestine and intestinal adenomas. The average number ( c ) and size ( d ) of macroscopic tumours observed in the small intestine of 13-week-old Apc min/− ; Vil-Cre TG/− ; RhoA DN/− animals and control Apc min/− ; Vil-Cre −/− ; RhoA DN/− mice are shown ( n =18). The average number ( e ) and size ( f ) of small intestinal tumours induced by AOM treatment in Vil-Cre −/− ;RhoA DN/− animals and Vil-Cre TG/− ;RhoA DN/− mice are shown. ( g , h ) Mice were i.p. injected with 100 mg kg −1 BrdU 2 h before being killed. The number of cells in the S-phase of the cycle during this time was assessed with anti-BrdU immunohistochemistry. ( i ) Pictures were taken under a bright-field microscope at × 20 and the number of proliferative cells in the small intestinal tumours of DN-RhoA ( Apc min/+ ;Vil-Cre TG/− ;RhoA DN/− ) and control ( Apc min/+ ;Vil-Cre −/− ;RhoA DN/− ) mice was quantified blinded from the animal identity. At least 1,000 total tumour cells were scored per mouse and there were seven mice per group. N : number of animals per group. The mean (±s.e.m.) is shown. *Student’s t -test P <0.05; n/s: not significant. Scale bars, 100 μm. Full size image RHOA and growth/differentiation of human colon cancer cells To investigate the molecular mechanisms of tumour suppression of RHOA in the intestine, we used four isogenic colon cancer cell line systems in which RHOA was inactivated by overexpression of a dominant negative mutant of RHOA (T19N) or RHOA-specific short hairpin RNAs (shRNAs; Supplementary Fig. 3 ). Reduced RHOA activity resulted in increased proliferation ( Fig. 2a–h and Supplementary Fig. 4a,b ) and anchorage-independent growth ( Fig. 2i–l and Supplementary Fig. 4c,d ) in all four cell line systems. Moreover, using a subcutaneous xenograft model we demonstrated that RHOA inactivation resulted in enhanced growth of colon cancer cells in vivo ( Fig. 2m,n and Supplementary Fig. 5 ), and this was associated with an increase in the number of proliferating cells (BrdU-positive) and a decrease in the number of apoptotic cells (active Caspase 3-positive; Fig. 2o–r ). 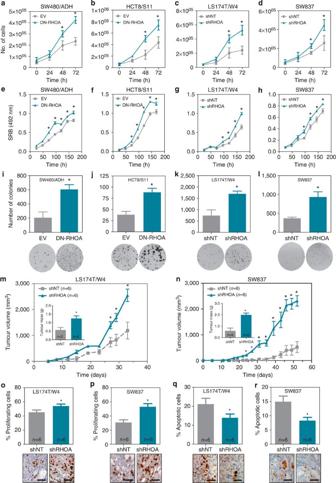Figure 2: Effects of RHOA inactivation on the growth of colorectal cancer cells. The effects of RHOA inactivation on the growth of SW480/ADH (a,e), HCT8/S11 (b,f), LS174T/W4 (c,g) and SW837 (d,h) colon cancer cells assessed as cell number (a–d) or SRB staining (e–h) are shown. Panelsi–lshow changes after RHOA inactivation in the growth of these four cell lines in soft agar. Changes in the growth of LS174T/W4 and SW837 cells after RHOA knockdown were assessed in a subcutaneous xenograft model (NOD/SCID mice;n=6). The inset inm,nshows the average tumour weight (±s.e.m.) at the end of the experiment. The average percentage (±s.e.m.) of proliferating (BrdU-positive;o–p) and apoptotic (active Caspase 3-positive;q–r) cells in the xenografts of LS174T/W4 (o,q) and SW837 (p,r) cells with and without RHOA inactivation is shown. The mean (±s.e.m.) of three independent experiments run in triplicate is shown. *Student’st-testP<0.05. Scale bars, 50 μm. Figure 2: Effects of RHOA inactivation on the growth of colorectal cancer cells. The effects of RHOA inactivation on the growth of SW480/ADH ( a , e ), HCT8/S11 ( b , f ), LS174T/W4 ( c , g ) and SW837 ( d , h ) colon cancer cells assessed as cell number ( a – d ) or SRB staining ( e – h ) are shown. Panels i – l show changes after RHOA inactivation in the growth of these four cell lines in soft agar. Changes in the growth of LS174T/W4 and SW837 cells after RHOA knockdown were assessed in a subcutaneous xenograft model (NOD/SCID mice; n =6). The inset in m , n shows the average tumour weight (±s.e.m.) at the end of the experiment. The average percentage (±s.e.m.) of proliferating (BrdU-positive; o – p ) and apoptotic (active Caspase 3-positive; q – r ) cells in the xenografts of LS174T/W4 ( o , q ) and SW837 ( p , r ) cells with and without RHOA inactivation is shown. The mean (±s.e.m.) of three independent experiments run in triplicate is shown. *Student’s t -test P <0.05. Scale bars, 50 μm. Full size image Members of the RHO family of small GTPases are known to be involved in the polarization of epithelial cells [35] , [36] , and we have recently shown that the loss of polarization and differentiation is important in the initial stages of intestinal tumorigenesis [34] . To investigate the role of RHOA in the polarization of colon cancer cells, we used LS174T/W4 cells with inducible LKB1 signalling, which upon doxycycline treatment display a fully polarized phenotype [37] . We found that induction of polarization was associated with an increase in the levels of GTP-bound active RHOA ( Fig. 3a ). To investigate whether this was the cause or effect of the polarization process, we blocked RHOA signalling in LS174T/W4 cells by either RHOA knockdown or treatment with the RHOA inhibitor exoenzyme C3 transferase. Reduced RHOA activity led to a significant reduction in the number of cells that were able to undergo polarization in response to LKB1 activation ( Fig. 3b and Supplementary Fig. 4e ), and this was dependent upon the RHOA effectors Rho-associated protein kinase (ROCK) and diaphanus-related formin 1 (DIAPH1), but not upon protein kinase N1 (PKN1) ( Fig. 3c–f ). Moreover, RHOA inactivation interfered with the capacity of colon cancer cells to differentiate after 21 days in confluent culture, as determined by the decreased activity of the enterocytic differentiation markers sucrose-isomaltase (SI), alkaline phosphatase (AP) and dipeptidyl peptidase 4 (DPP4; Fig. 3g–i ). In addition, using a cohort of 160 Dukes C colorectal cancer cases, we found that the levels of RHOA protein expression assessed by immunohistochemistry (IHC) with a RHOA-specific antibody ( Supplementary Fig. 5 ) [28] were significantly lower in poorly differentiated tumours compared with moderately/highly differentiated colorectal tumours ( Fig. 4 ), further indicating that RHOA regulates the differentiation of colorectal cancer cells. 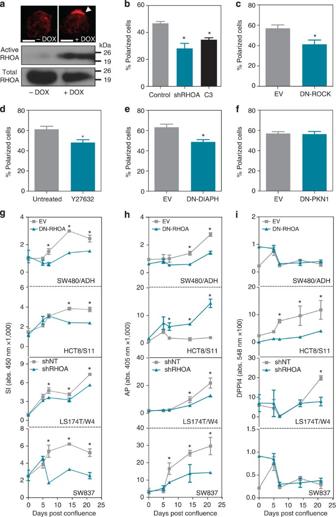Figure 3: Effects of RHOA inactivation on polarization and differentiation of colorectal cancer cells. (a) Activation of the LKB1/STRAD pathway by 24 h doxycycline (DOX) treatment in LS174T/W4 cells resulted in cell polarization, as revealed by the apical accumulation of actin (white arrowhead in the upper panel; rhodamine-phalloidin staining). The levels of active RHOA were determined by a GST-Rhotekin pull-down assay in nonpolarized and polarized LS174T/W4 cells (lower panel). Scale bars, 5 μm. (b) The average percentage of polarized LS174T/W4 cells was assessed after RHOA inhibition with shRHOA-TR10 or TAT-C3 transferase. (c–f) Average percentage of polarized LS174T/W4 cells after LKB1 activation and inhibition of the RHOA effectors ROCK, either with a dominant negative mutant (DN-ROCK) or the chemical inhibitor Y27632, DIAPH1 (DN-DIAPH1) or PKN1 (DN-PKN1). The effects of RHOA inactivation on the levels of activity of SI (g), AP (h) and DPP4 (i) were determined. The mean (±s.e.m.) of three independent experiments run in triplicate is shown. *Student’st-testP<0.05. Figure 3: Effects of RHOA inactivation on polarization and differentiation of colorectal cancer cells. ( a ) Activation of the LKB1/STRAD pathway by 24 h doxycycline (DOX) treatment in LS174T/W4 cells resulted in cell polarization, as revealed by the apical accumulation of actin (white arrowhead in the upper panel; rhodamine-phalloidin staining). The levels of active RHOA were determined by a GST-Rhotekin pull-down assay in nonpolarized and polarized LS174T/W4 cells (lower panel). Scale bars, 5 μm. ( b ) The average percentage of polarized LS174T/W4 cells was assessed after RHOA inhibition with shRHOA-TR10 or TAT-C3 transferase. ( c – f ) Average percentage of polarized LS174T/W4 cells after LKB1 activation and inhibition of the RHOA effectors ROCK, either with a dominant negative mutant (DN-ROCK) or the chemical inhibitor Y27632, DIAPH1 (DN-DIAPH1) or PKN1 (DN-PKN1). The effects of RHOA inactivation on the levels of activity of SI ( g ), AP ( h ) and DPP4 ( i ) were determined. The mean (±s.e.m.) of three independent experiments run in triplicate is shown. *Student’s t -test P <0.05. 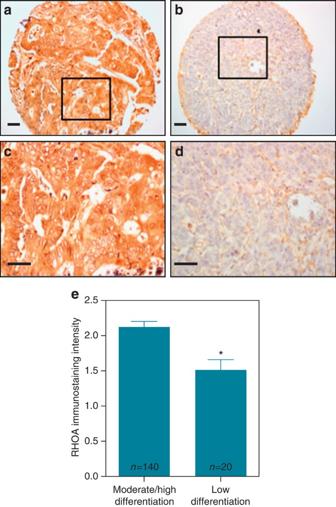Figure 4: RHOA expression in primary colorectal tumours with different degrees of differentiation. The levels of RHOA in 160 patients with Dukes C colorectal cancer were assessed by immunohistochemistry. Panelsa,bshow representative highly and poorly differentiated tumours, respectively. Higher magnification of the indicated areas is shown inc,d. Scale bars, 50 μm. The intensity of the RHOA immunostaining was quantified blinded from the clinical patient data. The histogram ineshows the average intensity (±s.e.m.) of RHOA immunostaining in tumours with low and moderate/high differentiation. *Student’st-testP<0.05. Full size image Figure 4: RHOA expression in primary colorectal tumours with different degrees of differentiation. The levels of RHOA in 160 patients with Dukes C colorectal cancer were assessed by immunohistochemistry. Panels a , b show representative highly and poorly differentiated tumours, respectively. Higher magnification of the indicated areas is shown in c , d . Scale bars, 50 μm. The intensity of the RHOA immunostaining was quantified blinded from the clinical patient data. The histogram in e shows the average intensity (±s.e.m.) of RHOA immunostaining in tumours with low and moderate/high differentiation. *Student’s t -test P <0.05. Full size image RHOA inactivation enhances Wnt/β-catenin signalling Since RHOA signalling has been shown to be necessary to maintain adherens junctions in normal epithelial cells and in colon cancer cells [15] , [38] , [39] , we investigated whether RHOA inactivation can modulate the levels of β-catenin involved in this structural role. Co-immunoprecipitation experiments demonstrated reduced levels of E-cadherin-bound β-catenin after RHOA inactivation in these cells ( Fig. 5a ). In the absence of a functional β-catenin destruction complex ( Supplementary Fig. 6 ), β-catenin was found to accumulate in the nucleus of colon cancer cells after RHOA inactivation ( Fig. 5b–j ). These findings raised the possibility that the redistribution of β-catenin from the membrane to the nucleus may enhance TCF4/β-catenin transcriptional activity. To test this we used a reporter assay containing wild-type or mutant TCF4/β-catenin-binding sites upstream of a luciferase reporter gene to assess changes in Wnt/β-catenin signalling. Inhibition of RHOA activity in colon cancer cells with either a dominant negative form of RHOA, targeted shRHOA knockdown or the RHOA inhibitor exoenzyme C3 transferase, each significantly increased the activity of TCF4/β-catenin ( Fig. 5k–m and Supplementary Fig. 7a,b ) as well as the activity of the transcription factor c-MYC, an important downstream target of TCF4/β-catenin ( Fig. 5n–p and Supplementary Fig. 7c,d ), and these effects were dependent on the RHOA effectors ROCK and DIAPH1, but not on PKN1 ( Fig. 6 ). Furthermore, RHOA inactivation in these four cell lines led to increased expression levels of c-MYC as well as other Wnt target genes, such as cyclin D1, Claudin 1 and LEF1 ( Fig. 7 ). 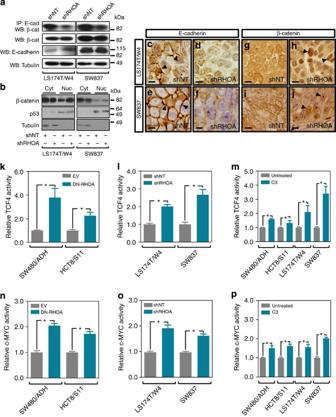Figure 5: Wnt and c-MYC activity after RHOA inactivation in colon cancer cells. (a) Total protein lysates from LS174T/W4 and SW837 stably transduced with a non-target shRNA (shNT) or shRHOA-TR10 (shRHOA) were immunoprecipitated with a mouse monoclonal anti-E-cadherin antibody and the levels of β-catenin interacting with E-cadherin assessed by western blotting. The total levels of β-catenin and E-cadherin are also shown and tubulin levels were used as a loading control. (b) Western blot showing β-catenin levels in cytoplasmic and nuclear protein fractions. (c–f) Immunohistochemistry of E-cadherin in subcutaneous xenografts of shNT control LS174T/W4 (c) and SW837 (e) cells or the corresponding RHOA knockdown cells (shRHOA;d,f, respectively). Arrowheads indicate membrane E-cadherin staining. (g–j) Immunohistochemical staining of β-catenin in subcutaneous xenografts of control LS174T/W4 (g) and SW837 (i) cells or the corresponding RHOA knockdown cells (shRHOA;h,j, respectively). Arrowheads indicate nuclear localization of β-catenin. Scale bars, 5 μm. (k–m) TCF4/β-catenin transactivation activity (TOP-FLASH/FOP-FLASH luciferase reporter) after RHOA inactivation with DN-RHOA (k), RHOA knockdown (shRHOA-TR10;l) or treatment with the chemical RHOA inhibitor TAT-C3 transferase (m). Panelsn–pshow changes in c-MYC transactivation activity (luciferase reporter assay) after RHOA inactivation with DN-RHOA (n), RHOA knockdown (o; shRHOA-TR10) or treatment with the chemical RHOA inhibitor TAT-C3 transferase (p). The mean (±s.e.m.) of three independent experiments run in triplicate is shown. *Student’st-testP<0.05. Figure 5: Wnt and c-MYC activity after RHOA inactivation in colon cancer cells. ( a ) Total protein lysates from LS174T/W4 and SW837 stably transduced with a non-target shRNA (shNT) or shRHOA-TR10 (shRHOA) were immunoprecipitated with a mouse monoclonal anti-E-cadherin antibody and the levels of β-catenin interacting with E-cadherin assessed by western blotting. The total levels of β-catenin and E-cadherin are also shown and tubulin levels were used as a loading control. ( b ) Western blot showing β-catenin levels in cytoplasmic and nuclear protein fractions. ( c – f ) Immunohistochemistry of E-cadherin in subcutaneous xenografts of shNT control LS174T/W4 ( c ) and SW837 ( e ) cells or the corresponding RHOA knockdown cells (shRHOA; d , f , respectively). Arrowheads indicate membrane E-cadherin staining. ( g – j ) Immunohistochemical staining of β-catenin in subcutaneous xenografts of control LS174T/W4 ( g ) and SW837 ( i ) cells or the corresponding RHOA knockdown cells (shRHOA; h , j , respectively). Arrowheads indicate nuclear localization of β-catenin. Scale bars, 5 μm. ( k – m ) TCF4/β-catenin transactivation activity (TOP-FLASH/FOP-FLASH luciferase reporter) after RHOA inactivation with DN-RHOA ( k ), RHOA knockdown (shRHOA-TR10; l ) or treatment with the chemical RHOA inhibitor TAT-C3 transferase ( m ). Panels n – p show changes in c-MYC transactivation activity (luciferase reporter assay) after RHOA inactivation with DN-RHOA ( n ), RHOA knockdown ( o ; shRHOA-TR10) or treatment with the chemical RHOA inhibitor TAT-C3 transferase ( p ). The mean (±s.e.m.) of three independent experiments run in triplicate is shown. *Student’s t -test P <0.05. 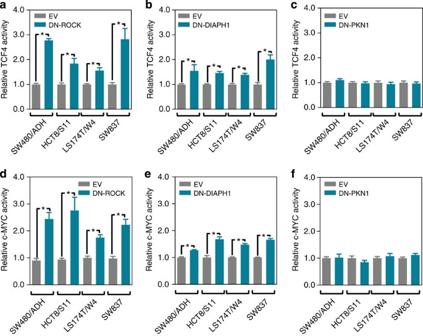Figure 6: Wnt and c-MYC activity after inhibition of the RHOA effectors ROCK, DIAPH1 and PKN1. Changes in TCF4/β-catenin activity (a–c) and c-MYC activity (d–f) after the RHOA effectors ROCK (a,d), DIAPH1 (b,e) and PKN1 (c,f) were inhibited with the corresponding dominant negative mutant forms. The mean (±s.e.m.) of three independent experiments run in triplicate is shown. *Student’st-testP<0.05. Full size image Figure 6: Wnt and c-MYC activity after inhibition of the RHOA effectors ROCK, DIAPH1 and PKN1. Changes in TCF4/β-catenin activity ( a – c ) and c-MYC activity ( d – f ) after the RHOA effectors ROCK ( a , d ), DIAPH1 ( b , e ) and PKN1 ( c , f ) were inhibited with the corresponding dominant negative mutant forms. The mean (±s.e.m.) of three independent experiments run in triplicate is shown. *Student’s t -test P <0.05. 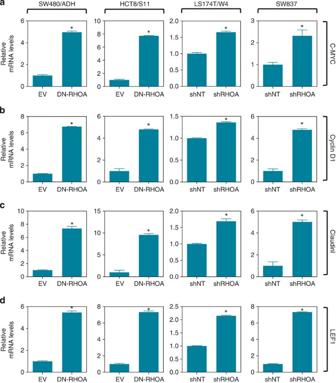Figure 7: Effects of RHOA inactivation on the expression of TCF4/β-catenin target genes. Changes in the levels of expression of the canonical Wnt/β-catenin target genes c-MYC (a), Cyclin D1 (b), Claudin I (c) and LEF1 (d) were assessed by real-time RT–PCR after RHOA inactivation with either a dominant-negative mutant of RHOA (DN-RHOA; SW480/ADH and HCT8/S11) or an shRNA against RHOA (shRHOA-TR10; LS174T/W4 and SW837). The mean (±s.e.m.) of three independent experiments carried out in triplicate is shown. *Student’st-test,P<0.05. Full size image Figure 7: Effects of RHOA inactivation on the expression of TCF4/β-catenin target genes. Changes in the levels of expression of the canonical Wnt/β-catenin target genes c-MYC ( a ), Cyclin D1 ( b ), Claudin I ( c ) and LEF1 ( d ) were assessed by real-time RT–PCR after RHOA inactivation with either a dominant-negative mutant of RHOA (DN-RHOA; SW480/ADH and HCT8/S11) or an shRNA against RHOA (shRHOA-TR10; LS174T/W4 and SW837). The mean (±s.e.m.) of three independent experiments carried out in triplicate is shown. *Student’s t -test, P <0.05. Full size image Consistent with these findings in vitro , microarray transcriptomic analysis of intestinal tumours from control ( Apc min/+ ;Vil-Cre −/− ;RhoA DN/− ) and DN-RhoA ( Apc min/+ ;Vil-Cre TG/− ;RhoA DN/− ) mice revealed a coordinated activation of canonical Wnt/β-catenin signalling in vivo . Using LS174T cells engineered to conditionally downregulate canonical Wnt signalling by doxycycline-dependent expression of either a dominant negative mutant of TCF4 (ref. 40 ) or a β-catenin-specific shRNA [41] , a core set of 281 genes regulated by β-catenin/TCF4 was defined. A significant inverse correlation was observed between the fold differences of these genes in control and doxycycline-treated dn-TCF4 LS174T cells and in tumours from control Apc min/+ and Apc min/+ mice expressing DN-RhoA (Spearman’s r =−0.2; P <0.001; Supplementary Table 1 ), indicating that RhoA inactivation further enhances β-catenin/TCF4 target gene expression. Of the 33,793 genes investigated, 1,268 (3.75%) showed significant expression differences in the tumours from control and DN-RhoA mice, including several known targets of Wnt/β-catenin signalling such as SOX2 and interleukin 6 ( Supplementary Table 2 ). Consistent with our findings in colon cancer cell lines, RhoA inactivation resulted in reduced levels of expression of multiple markers of differentiation, including AP 3, amylases 2a1 and 2a5 and lysozyme 1 ( Supplementary Table 2 ). In addition, gene-set enrichment analysis identified additional Gene Ontology categories that were significantly enriched in the number of genes differentially expressed, including G-protein-coupled receptor activity and extracellular space location ( Supplementary Table 3 ), suggesting additional mechanism contributing to the pro-tumorigenic phenotype observed after RhoA inactivation. Because RHOA has been shown to be an effector of noncanonical Wnt/PCP signalling [20] , we also investigated the effects of the non-canonical Wnt ligand Wnt5a on RHOA activity. As expected [42] , RHOA was activated in MDA-MB-231 breast cancer cells after Wnt5a treatment for 30 min ( Supplementary Fig. 8 ). In contrast, the levels of active RHOA did not significantly change after Wnt5a treatment in colon cancer cells ( Supplementary Fig. 8 ), suggesting that non-canonical Wnt signaling is not a major regulator of RHOA activity in colorectal cancer cells. To investigate to what extent the phenotypic changes observed after RHOA inactivation in colon cancer cells are dependent on the enhanced TCF4/β-catenin signalling, we restored TCF4/β-catenin activity back to the baseline levels observed in the control cells before blocking RHOA signalling. This was achieved in HCT8/S11 and SW837 cells with IWR-1, a potent chemical inhibitor of Wnt signalling [43] , and in LS174T cells by doxycycline-dependent expression of either a dominant negative mutant of TCF4 (ref. 40 ) or a β-catenin-specific shRNA [41] ( Fig. 8a ). Inhibition of the enhanced Wnt signalling in these cells completely recovered the proliferation ( Fig. 8b ) and the levels of differentiation ( Fig. 8c ) of the control cells with no RHOA inactivation, but had no effects on the polarization of LS174T cells after 2-deoxyglucose-treatment ( Fig. 8d ), a known inducer of polarization of these cells [44] . Therefore, we identified here a novel mechanism of deregulation of canonical Wnt signalling. In addition, reduced RHOA signalling also led to the loss of polarization of colon cancer cells through Wnt/β-catenin-independent mechanisms ( Supplementary Fig. 9 ). 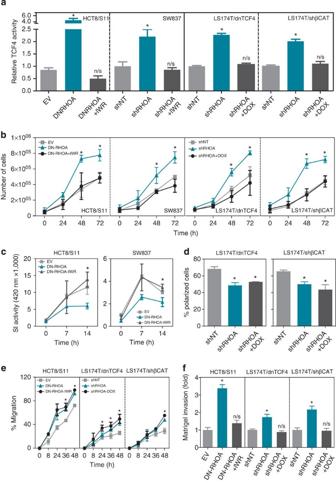Figure 8: TCF4/β-catenin signalling and proliferation, differentiation, invasion and motility of colon cancer cells after RHOA inactivation. (a) TCF4/β-catenin activity after inhibition of Wnt signalling with either IWR-1 (HCT8/S11 and SW837) or doxycycline-dependent expression of a dominant-negative mutant of TCF4 (LS174T/dnTCF4) or an shRNA against β-catenin (LS174T/shβCAT) in LS174T cells. The effects of TCF4/β-catenin inhibition on growth (cell number;b), differentiation (sucrase-isomaltase activity;c), 2-deoxyglucose-dependent polarization (d), motility (wound-healing assay;e) and matrigel invasion (Boyden chamber assay;f) of colon cancer cells is shown. The average (±s.e.m.) of three independent experiments run in triplicate is shown. *Student’st-testP<0.05. n/s: not significant. Figure 8: TCF4/β-catenin signalling and proliferation, differentiation, invasion and motility of colon cancer cells after RHOA inactivation. ( a ) TCF4/β-catenin activity after inhibition of Wnt signalling with either IWR-1 (HCT8/S11 and SW837) or doxycycline-dependent expression of a dominant-negative mutant of TCF4 (LS174T/dnTCF4) or an shRNA against β-catenin (LS174T/shβCAT) in LS174T cells. The effects of TCF4/β-catenin inhibition on growth (cell number; b ), differentiation (sucrase-isomaltase activity; c ), 2-deoxyglucose-dependent polarization ( d ), motility (wound-healing assay; e ) and matrigel invasion (Boyden chamber assay; f ) of colon cancer cells is shown. The average (±s.e.m.) of three independent experiments run in triplicate is shown. *Student’s t -test P <0.05. n/s: not significant. Full size image Loss of RHOA contributes to colon cancer metastasis We have previously shown that reduced RHOA levels are associated with lymph node metastasis in colorectal cancer patients [28] . To investigate the effects of RHOA inactivation on the metastatic potential of colon cancer cells, we first used the in vitro systems generated to assess changes in cell motility and invasion. RHOA inactivation led to significantly increased migration ( Fig. 9a–d and Supplementary Fig. 4f ) and matrigel invasion ( Fig. 9e–h ) in three of the four cell lines investigated. While the effect of the loss of RHOA on the motility of colon cancer cells was found to be Wnt-independent ( Fig. 8e ), the increased matrigel invasion capacity resulting from RHOA inactivation was fully dependent on the enhanced Wnt signalling observed ( Fig. 8f ). To directly address the role of RHOA in metastasis in vivo we used an experimental lung metastasis mouse model. When injected in the tail vein of immunodeficient nonobese diabetic/severe combined immunodeficiency (NOD/SCID) mice, SW837 and LS174T/W4 cells with RHOA inactivation formed more metastases than the corresponding control cells ( Fig. 9i ). The presence of lung metastases was confirmed on histological sections of the lungs of these animals ( Fig. 9j–l ). In good agreement, immunohistochemical staining of RHOA on sections from a tissue microarray containing paired primary tumour and distant metastasis samples from 26 Stage IV colorectal cancer patients revealed that the levels of RHOA were significantly reduced in distant metastases compared with the matched primary tumours ( Fig. 9m–p ). Collectively, these results demonstrate that RHOA inactivation significantly contributes to colorectal cancer metastasis. 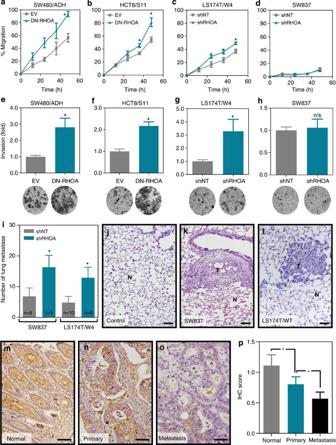Figure 9: Effects of RHOA inactivation on motility, matrigel invasion and metastasis of colon cancer. Changes in cell migration (a–d; wound-healing assay; percentage of wounded area closed after the indicated time), and matrigel invasion capacity (e–h; Boyden chamber invasion assay) after RHOA inactivation are shown. The mean (±s.e.m.) of three independent experiments run in triplicate is shown. (i) Average number (±s.e.m.) of macroscopically visible lung metastases after tail vein injection of control (shNT) and RHOA knockdown (shRHOA) SW837 and LS174T/W4 cells (n: number of mice per group). (j–l) Representative images of haematoxylin and eosin-stained histological sections from normal mouse lung (j) and metastatic lesions of SW837 (k) and LS174T/W4 (l) cells. N: normal; T: tumour. (m–o) Representative pictures of the levels of RHOA protein in paired normal mucosa (m), primary tumours (n) and distant metastases (o) as assessed by immunohistochemistry (Santa Cruz; SC-418). (p) Average intensity of the RHOA immunostaining (±s.e.m.) in the normal mucosa, primary tumours and distant metastases in a cohort of 26 advanced colorectal cancer cases. *Student’st-testP<0.05. Scale bars, 100 μm. Figure 9: Effects of RHOA inactivation on motility, matrigel invasion and metastasis of colon cancer. Changes in cell migration ( a – d ; wound-healing assay; percentage of wounded area closed after the indicated time), and matrigel invasion capacity ( e – h ; Boyden chamber invasion assay) after RHOA inactivation are shown. The mean (±s.e.m.) of three independent experiments run in triplicate is shown. ( i ) Average number (±s.e.m.) of macroscopically visible lung metastases after tail vein injection of control (shNT) and RHOA knockdown (shRHOA) SW837 and LS174T/W4 cells (n: number of mice per group). ( j – l ) Representative images of haematoxylin and eosin-stained histological sections from normal mouse lung ( j ) and metastatic lesions of SW837 ( k ) and LS174T/W4 ( l ) cells. N: normal; T: tumour. ( m – o ) Representative pictures of the levels of RHOA protein in paired normal mucosa ( m ), primary tumours ( n ) and distant metastases ( o ) as assessed by immunohistochemistry (Santa Cruz; SC-418). ( p ) Average intensity of the RHOA immunostaining (±s.e.m.) in the normal mucosa, primary tumours and distant metastases in a cohort of 26 advanced colorectal cancer cases. *Student’s t -test P <0.05. Scale bars, 100 μm. Full size image Canonical Wnt signalling is initiated in normal cells by the binding of Wnt ligands to receptors of the Frizzled and LRP families on the cell surface, and ultimately results in the disruption of the β-catenin destruction complex [18] , [45] . This results in elevated nuclear levels of β-catenin, which then binds to TCF/LEF transcription factors and regulates the transcription of the key mitogenic genes that orchestrate the tumorigenic process in colorectal cancer [17] , [18] . Constitutive activation of this pathway through mutations in APC or other genes involved in the β-catenin destruction complex are observed in the vast majority of colorectal tumours [19] . Noncanonical Wnt signalling is not as well understood but involves mechanisms independent of TCF/β-catenin transcriptional activity [20] . Although RHOA has previously been shown to participate in the noncanonical Wnt/PCP pathway both during embryogenesis and in some cancer types [46] , in colon cancer cells, RHOA activity did not change in response to the well-established noncanonical Wnt ligand Wnt5a, suggesting that noncanonical Wnt/PCP signalling is not a major regulator of RHOA in colorectal cancer cells. However, although the canonical Wnt/β-catenin signalling pathway has been extensively investigated for decades, the GTPase RHOA has not previously been shown to participate in this signalling cascade in cancer cells. Importantly, in addition to its activity as a transcriptional regulator, β-catenin plays a key structural role in the formation of the adherens junctions found in epithelial cells. The cytoplasmic domain of E-cadherin binds to α/β-catenin and to the actin cytoskeleton, thus stabilizing cell–cell junctions, and the binding of β-catenin to E-cadherin or TCF4 is mutually exclusive [39] . Consistent with earlier findings showing that RHOA signalling is necessary to maintain adherens junctions in normal intestinal epithelial cells and colorectal cancer cells [15] , [38] , RHOA inactivation in colon cancer cells was found to lead to reduced E-cadherin-bound β-catenin. Moreover, we found that RHOA inhibition results in the nuclear accumulation of β-catenin and further activates canonical Wnt signalling in colon cancer cells with elevated Wnt/β-catenin signalling due to APC (SW480/ADH, SW837 and HCT8/S11 cells) or CTNNB1 (β-catenin; LS174T cells) mutations. Consistently, increased Wnt/β-catenin signalling was observed also in the intestinal tumours of Apc min/+ mice after RhoA inactivation. This is in agreement with earlier studies showing that activation of Wnt/β-catenin signalling above the levels resulting from Apc min mutations can accelerate the tumorigenic process [47] , [48] , [49] . These results provide novel mechanistic insight into the deregulation of canonical Wnt signalling, a pathway of paramount importance in colorectal cancer and other tumour types. RHOA activation is generally considered to be oncogenic and to promote proliferation in different tissues [10] , [15] , [26] , [50] , [51] , [52] . Moreover, RHOA knockdown was reported to reduce the growth of colon cancer cells in a xenograft model [27] . However, canonical Wnt signalling has been shown to be a master regulator of proliferation of intestinal epithelial cells and colorectal tumours ‘hijack’ this important signalling pathway to maintain constant proliferation [40] , [53] . The further activation of TCF4/β-catenin activity imposed by the loss of RHOA in colon cancer cells would therefore be expected to result in increased proliferation and tumour growth. Indeed, using four different isogenic colon cancer cell line systems, we found that RHOA inactivation led to significantly faster growth in vitro and in vivo and this was shown to be dependent on ROCK/DIAPH-mediated activation of TCF4/β-catenin activity. Therefore, in colorectal tumours, the enhanced Wnt signalling resulting from the loss of RHOA, and the subsequent upregulation of multiple mitogenic proteins such as c-MYC and Cyclin D1, appears to compensate for any possible growth inhibitory effects induced by the loss of RHOA [51] , [52] . These results are consistent with earlier findings indicating that inhibition of ROCK signalling promotes the growth of colon cancer-initiating cells [54] . RHOA has been shown to be able to regulate polarization and differentiation through nontranscriptional signalling pathways [15] , [36] , [55] , [56] , [57] . However, Wnt signalling has also been shown to contribute to maintain an undifferentiated state in normal and transformed intestinal cells [58] , [59] . Here we show that Wnt signalling is important for the reduced levels of differentiation markers resulting from RHOA inactivation in colon cancer cells, and this is in agreement with the reported effects of TCF4/β-catenin on these enzymatic markers of enterocityc differentiation [58] . However, the reduced polarization observed after RHOA inactivation was found to be Wnt-independent. The apical differentiation of the intestinal epithelial cells known as the brush border is formed by a tight array of microvilli supported by a complex actin cytoskeleton. Previous studies have shown that RHOA can regulate the actin cytoskeleton of epithelial cells through Wnt-independent mechanisms mediated by its downstream effectors ROCK and DIAPH1 (refs 15 , 36 , 60 ). This is in agreement with our findings, suggesting that the observed effects of RHOA inactivation on cell polarization may be mediated through changes in actin and microtubule cytoskeleton dynamics. The results presented here indicate that the loss of RHOA in colon cancer cells orchestrates distinct features of enterocytic differentiation through different signalling pathways. Importantly, we found that reduced RHOA protein levels were associated with poorly differentiated tumours, which in turn correlates with poor prognosis of colorectal cancer patients. Similarly, the effects of RHOA inactivation on the motility of colon cancer cells likely involve the reorganization of the actin/microtubule cytoskeleton as well as changes in myosin activity, and/or cell–cell and cell–extracellular matrix adhesions [15] , [36] , [60] , although the detailed mechanisms remain to be fully elucidated. Recently, the loss of Cdc42, another member of the RHO GTPase family, has been shown to have a severe impact on the normal murine intestine, causing hyperplasia, abnormal Paneth cell differentiation and epithelial permeability [61] , although the contribution of these defects to intestinal tumorigenesis have not yet been investigated. Colorectal cancer mortality is largely attributed to the metastatic spread of the disease, and the molecular basis of this complex, multistage process is not fully understood [62] , [63] . Overexpression and activation of RHOA is widely believed to contribute to the metastasis process in multiple tumour types [13] , [14] , [64] , [65] , [66] . In intestinal tumours, RHOA activation with LPA has been shown to increase lymphatic invasion and peritoneal/pleural metastases in a rat model [24] . However, we have previously shown that reduced RHOA levels are associated with lymph node metastasis in colorectal cancer patients [28] . Here we show that targeted inactivation of RHOA significantly increases the motility and invasion of colon cancer cells in vitro and, using a mouse model of experimental metastasis, we demonstrate that the loss of RHOA significantly contributes to the metastatic spread of colon cancer cells in vivo . Importantly, we also found that distant metastases express lower levels of RHOA compared with matched primary human colorectal tumours. These results indicate that the small GTPase RHOA may have opposite effects in different tumour types, thus contributing to tumour metastasis in some tissues such as breast and ovarian cancer [64] , [65] , [66] , while suppressing the spread of colorectal tumours. In conclusion, we have identified a novel mechanism of activation of canonical Wnt signalling, a pathway universally deregulated in colorectal cancer. Moreover, we demonstrate that the elevated TCF4/β-catenin activity resulting from RHOA inactivation above the high levels because of APC or CTNNB1 mutations leads to increased proliferation, invasion and de-differentiation of colon cancer cells. In addition, RHOA inactivation also resulted in Wnt/β-catenin-independent increased motility and reduced ROCK/DIAPH1-dependent polarization of colon cancer cells. Using animal models we demonstrate that targeted inactivation of intestinal RhoA led to shorter survival and increased tumour burden after genetic or pharmacological initiation of intestinal tumorigenesis. Moreover, we show that the loss of RHOA is an important event contributing to colon cancer metastasis. Despite the oncogenic activity of RHOA in other tumour types, this study constitutes the first demonstration of the tumour and metastasis suppressor role of RHOA in colorectal cancer and highlights the divergent role of RHO GTPases in the tumorigenic process of different organs. Inhibition of RHO and ROCK is currently being investigated as a therapeutic approach for the treatment of cancer [67] , [68] . These results emphasize that caution should be taken when generalizing options for therapeutic intervention based on results obtained in other tumour types. Cell lines LS174T/W4 cells expressing inducible STRAD/LKB1 (ref. 37 ), LS174T/dnTCF4 with inducible dominant negative TCF4 expression [40] , LS174T/siβCAT with inducible expression of a β-catenin-specific shRNA [41] were a kind gift of Dr Hans Clevers (Hubrecht Laboratory and Centre for Biomedical Genetics, Utrecht, the Netherlands). SW480/ADH cells expressing an HA-tagged T19N dominant negative mutant of RHOA (DN-RHOA) [57] were a kind gift of Dr Alberto Muñoz (Instituto de Investigaciones Biomédicas Alberto Sols, Consejo Superior de Investigaciones Cientificas-Universidade Autónoma de Madrid, Madrid, Spain). HCT8/S11 cells expressing the T19N dominant negative mutant of RHOA were a kind gift of Dr Marc Mareel (Laboratory of Experimental Cancerology, Department of Radiotherapy and Nuclear Medicine, Ghent University Hospital, Ghent, Belgium). MDA-MB-231 cells were from American Type Culture Collection. Control L and L-Wnt3a cells were a kind gift of Dr Hector Palmer (Vall d’Hebron Institute of Oncology, Spain). Wnt5a cells were a kind gift of Dr Ron Smits (Erasmus MC University Medical Center Rotterdam, the Netherlands). After control L-cells or Wnt3a/wnt5a-expressing derivative cells reached 100% confluence, they were given fresh medium. Four days later, the conditioned medium was centrifuged and the supernatant filtered through a 45-μm filter. When indicated, cells were treated with 40 mM LiCl (Sigma) for 6 h, a 1:1 mix of Wnt3a-conditioned medium for 6 h or with a 1:1 mix of Wnt5a-conditioned media and fresh medium for 30 min. All cell lines used in this study were maintained on Dubelcco’s Modified Eagle’s Medium (SW837, SW480/ADH, HEK293T, MDA-MB-231 and L-cells; Sigma) or RPMI (LS174T/W4 and HCT8/S11; Sigma) containing 10% fetal bovine serum (Sigma) and 1 × antibiotic antimycotic (Life Technologies) at 37 °C/5% CO 2 . Clinical samples Primary colorectal tumour samples were collected at collaborating medical institutions in Spain, Finland and Australia. Written informed consent for genetic analysis of the tumour sample was obtained from each patient, according to protocols approved by the Human Investigations and Ethical Committee in the appropriate Institution. For tissue microarray preparation, areas containing a high proportion of tumour cells were selected after histological examination of H&E-stained tumour sections. Triplicate 0.6-mm cores from every sample were arrayed in a fresh paraffin block using a Beecher Instrument tissue arrayer (Silver Spring, MD). Unstained 4-μm sections from the tissue microarray were mounted on slides coated with 3-aminopropyl-triethoxy-silane (Sigma, St Louis, MO). Reagents TAT-C3 is a cell-permeable form of the RHOA inhibitor C3 transferase, which induces ADP-ribosylation and consequent inhibition of RHOA. To prepare TAT-C3, BL21(DE3)-pLys S bacteria were transformed with pGEX-KG TAT-MYC-C3. Expression of TAT-MYC-C3 was induced with 100 μM IPTG for 3 h at 37 °C. Cells were then pelleted trough centrifugation and resuspended in 10 ml of TBS lysis buffer (137 mM NaCl, 5 mM KCl, 25 mM Tris-HCl, pH 7.4, 1 mM dithiothreitol (DTT) and 1 mM phenylmethylsulphonyl fluoride). Lysates were disrupted with three 1-min rounds of sonication at 20% intensity using an MSE Soniprep 150, followed by the removal of debris by centrifugation at 10,000 g for 20 min at 4 °C. Clarified supernatants were incubated with 0.5 ml glutathione-Sepharose (GE Healthcare) bead slurry for 2 h at 4 °C to bind glutathione S-transferase (GST) fusion protein. Beads were washed three times with TBS lysis buffer, followed by two washes with thrombin cleavage buffer (1 mM MgCl 2 , 1 mM CaCl 2 , 1 mM DTT in TBS), resuspended in 0.5 ml of thrombin cleavage buffer and incubated overnight at 4 °C with 25 units of thrombine (Sigma) allowing for the release of TAT-MYC-C3 from the GST moiety. After incubation, the supernatant was removed, beads were washed twice with 0.5 ml thrombin cleavage buffer and the collected supernatants were incubated with 30 μl of TBS-washed p-aminobenzamide beads (Sigma) for 1 h to remove thrombin before snap-freezing aliquots, which were then stored at −80 °C.TAT-C3 toxin was added to the media (80 nM) and cells were treated for 24 h. Y27632 (Tocris Bioscience) a selective ROCK inhibitor was added to the cells at 10 μM for 24 h. The Wnt inhibitor IWR-1 (Sigma) [43] was used at a working concentration of 2.5 μM for the indicated time. Plasmids and stable RHOA downregulation pVSV-G, pCMV-dR8.91, pLKO-shRHOA (TRCN0000047710, TRCN0000047711 and TRCN0000047712; hereafter named TR10, TR11 and TR12, respectively) and pLKO-shNT shRNA (SHC016-1EA; all from Mission shRNA system, Sigma) were used to generate cell lines with stable downregulation of RHOA according to the manufacturer’s recommendations RHOA inhibition was tested by western blot using a RHOA antibody (1:1,000 Cytoskeleton, clone ARH03). M50 Super 8 × TOP-Flash (Addgene plasmid 12456) and M51 Super 8 × FOP-Flash (Addgene plasmid 12457) TCF4/β-catenin luciferase reporter plasmids, containing seven wild-type or mutated TCF/LEF-1-binding sites, respectively, upstream of a minimal TA viral promoter driving luciferase expression, a kind gift of Dr Randall Moon, were used to assess TCF4/β-catenin activity (Howard Hughes Medical Institute, Chevy Chase, MD, USA). The following vectors used have been described before: pEF-BOS-myc-ROCK-RB/PH-TT (DN-ROCK) expressing a dominant negative mutant of ROCK1 was a kind gift from Dr Kozo Kaibuchi (Department of Cell Pharmacology, Nagoya University Graduate School of Medicine, Nagoya, Japan); pEF-DIAPH1-ΔNΔC, a dominant negative mutant of DIAPH1 (DN-DIAPH1) unable to organize microtubules or promote actin polymerization [15] , was a kind gift from Dr Eric Sahai (London Research Institute, London, UK); pGEX-KG-TAT-MYC-C3, encoding a cell-permeable form of C3 transferase, was a gift from Dr Mike Olson (The Beatson Institute for Cancer Research, Glasgow, UK); pRC/CMV-FLAG-PKN1-K644E (DN-PKN1), containing the full coding sequence of PKN1 with the K644E dominant negative mutation, was a gift from Dr Hideyuki Mukai (Biosignal Research Center, Kobe University, Japan); luciferase reporter plasmids for c-MYC activity pBV-Luc WT-MBS1-4 (Addgene plasmid 16564), containing wild-type c-MYC-binding sites, and the respective mutated control pBV-Luc MUT-MBS1-4 (Addgene plasmid 16565) containing mutated c-MYC-binding sites, were a gift from Dr Bert Vogelstein (Howard Hughes Medical Institute, The Johns Hopkins Oncology Center, The Johns Hopkins University School of Medicine, Baltimore, MD, USA); pRL-TK expressing Renilla luciferase and pGL3-Basic were obtained from Promega. RHOA activity assay A GST-Rhotekin-RBD pull-down assay was used for the determination of RHOA activity with the RHO Activation Assay Biochem kit (Cytoskeleton) according to the manufacturer’s protocols. Proliferation, migration, invasion and soft-agar assays Proliferation was determined by cell counting and with the Sulforhodamine B (SRB) protein staining method. In brief, 2,000 cells were seeded on a 96-well microtitre plate (eight replicates per cell line). One plate was fixed with 10% TCA every 24 h for 6 days. Fixed plates were then stained with 0.4% SRB in 1% acetic acid for 30 min and then washed with 1% acetic acid. SRB precipitates were then dissolved in 10 mM Tris pH 10 and absorbance was measured at 590 nm. Absorbance measurements were plotted versus time and used to assess the cell density. To investigate changes in cell motility and invasion after RHOA downregulation, a wound-healing assay and a Boyden chamber assay were used. For the wound-healing assay, cell lines were seeded in six-well plates and allowed to grow until they reached 90% confluence (2 × 10 6 cells per well of each cell line). The cell monolayer was scratched with a sterile micropipette tip and the wound region was allowed to heal by cell migration. The area that remained clear of cells after 12, 24 and 48 h was quantified with Image J (National Institutes of Health) and compared with the area of the wound at time zero. For the invasion, a 24-well Boyden chamber (Beckton Dickinson; 8 μm pore size) covered with 100 μl of 1 mg ml −1 Matrigel (Beckton Dickinson) was used. Colon cancer cells were seeded at different densities (4 × 10 4 of SW480/ADH, 3 × 10 4 of HCT8/S11, 6 × 10 4 of LS174T-W4 and SW837 cells) in 100 μl of cell culture medium containing 1% fetal bovine serum (FBS) in the upper compartment of the transwell. The lower compartment was filled with culture medium with 10% FBS, acting as an attractant. After incubation for 48 h at 37 °C in 5% CO 2 , the cells that were unable to penetrate the filter were wiped out with a cotton swab, whereas the cells that had invaded the lower surface of the filter were fixed and stained with 5% crystal violet. The total number of invading cells was determined under the microscope ( × 10). A soft-agar assay was used to determine the anchorage-independent growth capability of the stable models. Cells (1 × 10 5 ) were resuspended in complete medium containing 0.3% agar and then plated on six-well plates on top of 0.6% agar in complete medium. Cultures were maintained at 37 °C in a 5% CO 2 incubator for 21 days. Colonies were then stained with nitro blue tetrazolium chloride (1 mg ml −1 ; Sigma) and the number of macroscopically visible colonies was scored. Xenograft and lung metastasis model All animal experiments were carried out under protocols approved by the Institutional Ethical Committee and the appropriate governmental agency. For the subcutaneous xenograft model , six NOD/SCID mice (Harlan Laboratories; six animals per group) were injected subcutaneously with 3 × 10 6 LS174T/W4-shNT (left flank) and LS174T/W4-shRHOA-TR10 (right flank) cells in 100 μl of PBS. The same experimental set-up was used for the SW837-shRHOA derivative line and the corresponding non-target shRNA control (1.5 × 10 6 cells). A caliper was used to monitor tumour growth over time. To study lung metastasis , 1.5 × 10 6 SW837-shNT or SW837-shRHOA-TR10 cells or 3 × 10 6 LS174T/W4-shNT or LS174T/W4-shRHOA-TR10 cells in 100 μl PBS were injected into the tail vein of athymic NOD/SCID mice (Harlan Laboratories; 10 animals per group). Animals injected with SW837 or LS174T/W4 cells were killed after 12 or 6 weeks, respectively, and their lungs were perfused with 4% formalin and fixed overnight. The number of macroscopically visible tumours was scored under a dissecting microscope (OLYMPUS SZH stereo-zoom microscope, magnification × 7.5). Samples were then embedded in paraffin, sectioned and stained with haematoxylin and eosin. Enzymatic activity assays Determination of the activity of the intestinal differentiation markers AP, SI and DPP4 in colon cancer cells was performed. For AP activity, 50 μg of protein (in a volume of 50 μl of mannitol buffer: (50 mM D-mannitol, 2 mM Tris and 0.1% Triton X-100)) were mixed with 200 μl of p-Nitrophenyl Phosphate Liquid Substrate System (Sigma N7653), incubated at 37 °C for 15 min and the absorbance was measured at 405 nm. For SI activity assay, 25 μg of protein in 12.5 μl of mannitol buffer were incubated with 12.5 μl of substrate (0.056 M maltose in mannitol buffer, pH 6.0) at 37 °C for 60 min. The reaction was stopped by heating at 100 °C for 2 min and the formed precipitate was resuspended in 250 μl of TGO buffer (horseradish peroxidase 5 mg, glucose oxidase 4 mg, o-dianisidine 10 mg and 0.2% Triton X-100 in a final volume of 100 ml of Tris 0.5 M, pH 7.0) and the absorbance measured at 450 nm. For DPP4 activity assay, 50 μg of protein in 90 μl of mannitol buffer were added to 10 μl of 1.4 M glycine-NaOH pH 8.7 and incubated in the presence of 100 μl of substrate (glycyl-L-proline-p-nitroanilide, final 1.5 mM) at 37 °C for 30 min. The reaction was stopped with 800 μl of 32% trichloroacetic acid and the samples were centrifuged at 1,700 r.p.m. for 10 min. Then, 50 μl of supernatant were added to 50 μl of cold 0.2% sodium nitrite and incubated at 4 °C for 10 min. Next, 50 μl of 0.5% ammonium sulfamate were added and, after 2 min of incubation, 100 μl of 0.05% n-(1-naphthyl)-ethanediamine were added and incubated at 37 °C for 30 min in the dark. The absorbance was read at 548 nm. Mouse strains C57BL/6J-Apc min /J mice were obtained from The Jackson Laboratory (Maine, USA). These mice carry the heterozygous inactivating mutation T2549A in the tumour-suppressor gene Apc . The C57BL/6J -CAT- RhoA -DN/4-18 mice carrying the cytomegalovirus promoter fused to a CAT gene cassette flanked by loxP sites and the dominant negative T19N mutant of RhoA [31] was obtained from the Riken Institute (CAT-RhoA DN/4-18; Tokyo, Japan). The B6.SJL-Tg(Vil-cre)997Gum/J mice hemizygous for the Villin-Cre transgene expressing Cre recombinase under the control of the Villin 1 promoter ( Vil-Cre TG/ ) [69] were obtained from the Jackson Laboratory. Mice carrying the inducible DN-RhoA were crossed with animals carrying Villin-Cre , resulting in intestine-specific expression of DN-RhoA . To initiate tumorigenesis in the intestine of the animals, Vil-Cre TG/− ;RhoA DN/− female animals were crossed with male Apc min/+ mice. As an alternative method to initiate intestinal tumorigenesis, 9-week-old Vil-Cre −/− : RhoA DN/− and Vil-Cre TG/− ; RhoA DN/− mice (both Apc +/+ ) were i.p. injected with the intestine-specific carcinogen AOM (10 mg kg −1 ) weekly for 9 weeks and killed 10 weeks after the last AOM injection. Histology and IHC The intestine of 13-week-old mice was dissected and fixed in 4% formalin. The number and size of macroscopically visible tumours was scored under a dissecting microscope (OLYMPUS SZH stereo-zoom microscope, magnification × 7.5) before paraffin inclusion. For IHC, the NovoLink polymer detection system (Novocastra Laboratories) was used. For assessment of proliferation, animals were i.p. injected with 100 mg kg −1 BrdU 2 h before being killed and the number of cells in S-phase was determined by anti-BrdU immunostaining (Developmental Studies Hybridoma Bank) following antigen retrieval with 10 mM citrate buffer pH 6.0. For assessment of apoptosis, the percentage of active Caspase 3-positive cells was determined (antigen retrieval in 1 mM EDTA, pH9.0 at 95 °C for 20 min; AF835; R&D Biosystems; 1:500). RHOA immunostaining was carried out with mouse monoclonal anti-RHOA (Santa Cruz; SC-418; 1:500) as previously described [28] . RHOA staining levels were scored in a semiquantitative scale from 0 (absence of RHOA immunostaining) to 3 (highest immunostaining). E-cadherin and β-catenin immunostaining was carried out after antigen retrieval with 10 mM citrate buffer pH 6.0 (BD Transduction; 610181 and 610154, respectively; both used at a 1:100 dilution). Microarray experiments Formalin-fixed, paraffin-embedded sections (10 μm) of the small intestine of control mice ( Apc min/+ ;Vil-Cre −/− ;RhoA DN/− ) and DN-RhoA-expressing animals ( Apc min/+ ;Vil-Cre TG/− ;RhoA DN/− ) were mounted on PEN membrane-covered microscope slides (Carl Zeiss Microscopy) and deparaffinized. Tumours from six animals per group (control and DN-RhoA ; average 5.25 tumours per animal) were macrodissected under a dissecting microscope (SHZ; Olympus). The tumours from three animals were pooled and total RNA extracted using the RNeasy Micro Kit (Qiagen) after protease K treatment (500 μg ml −1 ) for 15 min at 56 °C and then at 80 °C for 15 min. Total RNA was amplified using the Complete Whole Transcriptome Amplification Kit (Sigma), labelled using the Mapping 250K NSP Assay kit (Affymetrix) and hybridized to Mouse Gene 2.1 ST arrays (total of 4 arrays; Functional Genomics Core, Institute for Research in Biomedicine, Barcelona). Expression data were Robust Multi-array Average (RMA)-normalized and, to assess the level of background variability between hybridizations, we examined the mean fold difference of 78 housekeeping genes [70] in tumours from control and DN-RhoA animals and it was found to be 0.97±0.13 (mean±s.d.). The 1,268 genes with expression differences greater than two times the s.d. observed for these housekeeping genes (0.97±0.26; mean±2 × s.d.) in tumours from control and DN-RhoA mice were considered to be differentially expressed. Gene-set enrichment analysis using Gene Ontology terms was carried out using DAVID Bioinformatics Resources 6.7. A core set of 281 genes regulated by Wnt signalling in colon cancer cells was identified using expression microarray data from LS174T cells where Wnt signalling is downregulated by the overexpression of a dominant negative form of TCF4 or an shRNA against β-catenin [40] , [41] (genes with more than twofold expression difference in control and Doxycycline-treated cells and a Student’s t -test P <0.05). Data available at Gene Expression Omnibus ID: GDS4386. Luciferase reporter assays To assess TCF4/β-catenin activity, we co-transfected 10 ng Renilla luciferase plasmid (pRL-TK; Promega) and 50 ng of either TOP-flash or FOP-flash luciferase reporter plasmids using Lipofectamine 2000 (Invitrogen). Firefly and Renilla luciferase activities were measured using the Dual-Luciferase assay Kit (Promega) with a FB-12 luminometer (Berthold). When indicated, cells were treated with permeable TAT-C3 transferase (80 nM) for 24 h or co-transfected with DN-ROCK, DN-DIAPH1, DN-PKN1 or the corresponding empty vector controls. For determination of c-MYC promoter activity, the luciferase reporter plasmids pBV-Luc WT-MBS1-4 and pBV-Luc MUT-MBS1-4 were used. Cytoplasmic and nuclear protein extracts and western blotting For cytoplasmic and nuclear protein fractionations, cell pellets were resuspended in cytoplasmic extraction buffer (1 M HEPES; 2 M KCl, 0.5 M EDTA 0.3% NP-40 and protease inhibitors) and incubated 5 min on ice. Lysates were centrifuged for 5 min at 3,000 r.p.m. at 4 °C and supernatants were collected as cytoplasmic extract. Remaining pellets were washed twice with 100 μl of cytoplasmic extraction buffer without NP-40 and then resuspended in an equal volume of nuclear extraction buffer (1 M HEPES; 5 M NaCl; 0.5 M EDTA; 25% Glycerol and protease inhibitors). Lysates were incubated on ice for 10 min and then centrifuged for 5 min at 4 °C 12,000 r.p.m. The collected supernatant was stored as nuclear extract. Western blotting was carried out as previously described [34] using total protein extracts or nuclear/cytoplasmic fractions as indicated. The antibodies used were: mouse monoclonal anti-p53 antibody (OP43; Calbiochem; 1:500); mouse monoclonal anti-β-tubulin antibody (T4026; Sigma; 1:2,500); anti-mouse monoclonal anti-RHOA antibody (ARH03; Cytoskeleton; 1:1,000); mouse monoclonal anti-β-catenin antibody (610154; BD Transduction; 1:1,000). Full-length images of immunoblots are shown in Supplementary Fig. 10 . Immunoprecipitation analysis Confluent cells in 10-cm tissue culture dishes were washed in PBS containing 10 mM CaCl 2 , then lysed in 1 ml lysis buffer (1% NP-40, 1% Triton X-100, 50 mM Tris-HCl, pH 7.4, 100 mM NaCl, 5 mM CaCl 2 and protease inhibitors) and incubated on ice for 30 min in rotation before clearing by centrifugation at 14,000 r.p.m. for 5 min. The supernatant was incubated with a mouse monoclonal anti-E-cadherin antibody (5 μg, Clone 36; BD Biosciences) and Protein G PLUS Agarose (40 μl, Santa Cruz). Following overnight incubation at 4 °C, immunocomplexes were collected and washed three times (0.05% NP-40, 50 mM Tris-HCl, pH 7.4, 0.5 M NaCl). Beads were resuspended in 30 μl of Laemmli buffer and analysed by SDS–PAGE and immunoblotted with an anti-β-catenin antibody as described above. Polarization assay For quantification of polarized LS174T/W4, cells were seeded on gelatin-coated glass coverslips and transfected (Lipofectamine 2000, Invitrogen) with DN-ROCK, DN-DIAPH1 or DN-PKN1 when applicable. Twenty-four hours after transfection, cell polarization was induced by activating the STRAD-LKB1 pathway with 5 μg ml −1 doxycycline (Sigma [37] ) and treated with Y27632 when indicated. Polarization of LS174T/dnTCF4 and LS174T/siβCAT cells and derivative shRHOA-overexpressing cells was assessed after 1 h of serum starvation and 2 h treatment with 50 mM 2-deoxyglucose [44] . Cells were then fixed in 4% paraformaldehyde, permeabilized with 0.1% Triton X-100 and stained with rhodamine-phalloidin (0.1 μM; Cytoskeleton). Polarization was scored using a fluorescent microscope (Olympus BX61 equipped with a DP70 camera). Polarized cells were defined by the characteristic accumulation of actin in one pole of the cell as previously described [34] , [37] , [44] . At least 500 polarized and unpolarized cells were scored blinded from the sample ID in three independent experiments. Quantitative RT–PCR Cell cultures were harvested at 70% confluence and total RNA was extracted using TRI Reagent (Molecular Research Center) according to the manufacturer’s instructions. Total RNA (500 ng) was reverse-transcribed using the High Capacity cDNA Reverse Transcription kit (Applied Biosystems, Branchburg, NJ), and relative levels of the indicated genes were assessed by Real-Time PCR using SYBR Green Master Mix (Applied Biosystems). PCR primers The primers used were as follows: c-MYC (forward primer 5′-CAGCTGCTTAGACGCTGGATT-3′; reverse primer 5′-GTAGAAATACGGCTGCACCGA-3′), Cyclin D1 (forward primer 5′-GCGGAGGAGAAACCAGAT-3′; reverse primer 5′-TGAACTTCACATCTGTGGCA-3′), claudin1 (forward primer 5′-CCCTATGACCCCAGTCAATG-3′; reverse primer 5′-ACCTCCCAGAAGGCAGAGA-3′) and Lef1 (forward primer 5′-AGAACACCCCGATGACGGA-3′; reverse primer 5′-GGCATCATTATGTACCCGGAAT-3′). Mouse genotyping was performed with DNA prepared from the mouse ear. Specific primers for RhoA dominant negative mutant (forward primer 5′-CTCATAGTCTTCAGCAAGGACCAGTT-3′; reverse primer 5′-ATCATTCCGAAGATCCTTCTTATT-3′), Apc (forward primer 5′-TTCCACTTTGGCATAAGGC-3′; reverse primer for the wild-type allele 5′-GCCATCCCTTCACGTTAG-3′; reverse primer for the mutated allele 5′-TTCTGAGAAAGACAGAAGTTA-3′) and Vil -CRE (forward primer 5′-CAAGCCTGGCTCGACGGCC-3′; reverse primer 5′-CGCGAACATCTTCAGGTTCT-3′) were used. For determination of correct Cre recombination in the DN-RhoA/Vil-CRE mice , total RNA prepared from the intestine of double transgenic mice was reverse transcribed and analysed by PCR amplification with DN-RhoA primers and Cat primers (forward primer 5′-CAGTCAGTTGCTCAATGTACC-3′; reverse primer 5′-ACTGGTGAAACTCACCCA-3′). The size of amplified DNA was 390 bp for Cat and 617 bp for DN-RhoA. Accession codes: ArrayExpress ID: E-MTAB-2981. How to cite this article : Rodrigues, P. et al. RHOA inactivation enhances Wnt signalling and promotes colorectal cancer. Nat. Commun. 5:5458 doi: 10.1038/ncomms6458 (2014).